Transformation of the intestinal epithelium by the MSI2 RNA-binding protein The MSI2 RNA-binding protein is a potent oncogene playing key roles in haematopoietic stem cell homeostasis and malignant haematopoiesis. Here we demonstrate that MSI2 is expressed in the intestinal stem cell compartment, that its expression is elevated in colorectal adenocarcinomas, and that MSI2 loss-of-function abrogates colorectal cancer cell growth. MSI2 gain-of-function in the intestinal epithelium in a drug-inducible mouse model is sufficient to phenocopy many of the morphological and molecular consequences of acute loss of the APC tumour suppressor in the intestinal epithelium in a Wnt-independent manner. Transcriptome-wide RNA-binding analysis indicates that MSI2 acts as a pleiotropic inhibitor of known intestinal tumour suppressors including Lrig1, Bmpr1a, Cdkn1a and Pten. Finally, we demonstrate that inhibition of the PDK–AKT–mTORC1 axis rescues oncogenic consequences of MSI2 induction. Taken together, our findings identify MSI2 as a central component in an unappreciated oncogenic pathway promoting intestinal transformation. The Drosophila melanogaster RNA-binding protein Musashi contributes to asymmetric stem cell division and cell fate determination in the neuroblast [1] . In mammals, there are two Musashi orthologues, MSI1/Msi1 and MSI2/Msi2 (ref. 2 , 3 ). Recently, Msi2 has been implicated as a critical regulator of haematopoietic stem cell (HSC) self-renewal and fate determination and MSI2 is a potent cooperative oncogene in human leukaemias [4] , [5] , [6] . The role of MSI2 in leukaemia progression was recently revealed by two groups who independently observed increased MSI2 expression during disease progression in patients with chronic myelogenous leukemia (CML) blast crisis and in acute myeloid leukaemias [4] , [5] . Forced MSI2 expression drove a more aggressive myeloid disease in a transplantation model utilizing the BCR-ABL oncogene. In contrast, MSI2 abrogation in myeloid leukaemia cells increases differentiation, decreases proliferation and increases apoptosis [4] . These studies demonstrate that MSI2 cooperates with known oncogenes in haematopoietic malignancies. In addition, high MSI2 expression is observed in a variety of other cancers, including hepatocellular carcinoma and lung cancer [7] , [8] , suggesting an important role for MSI2 in a variety of epithelial-derived carcinomas. Aggressive leukaemias are characterized by the prevalence of an increasingly HSC-like transcriptional profile. Consistent to the role of MSI2 in leukaemia, MSI2 also plays an important role in HSC homeostasis. MSI2 is highly expressed in the most primitive HSCs, including long-term HSCs and short-term HSCs, but not in more committed haematopoietic lineages. Inactivation of Msi2 in HSCs impairs their competitive repopulation ability upon transplantation [4] , [6] , [9] . Thus, although the functions of MSI2 in normal and malignant haematopoiesis are well established, little is known regarding the role MSI2 plays in stem cells and cancers in other organ systems. In contrast to reports of MSI2 function in the haematopoietic system, several reports have suggested a role for the second Musashi family member, MSI1 in colorectal cancer (CRC). Msi1 is expressed in the putative intestinal stem cell (ISC) compartment [10] and overexpressed in colorectal adenocarcinoma, where higher expression level of MSI1 is correlated to increased metastatic risk and poorer survival [11] , [12] . The putative role of MSI1 in CRC and ISCs, coupled with our past observations of MSI2 function in the HSC and haematopoietic cancers, prompted us to investigate a role of MSI2 in intestinal transformation. CRC is one the leading causes of cancer-related deaths globally. Genetic inactivation of the adenomatous polyposis coli ( APC ) tumour suppressor gene is believed to initiate the majority of human CRCs, and elegant genetic studies suggest that APC loss only initiates tumorigenesis when it occurs in ISCs with self-renewal capacity [13] . APC loss drives constitutive activity of the canonical Wnt signalling pathway by preventing the degradation of its downstream transcriptional effector β-catenin. Thus, constitutive β-catenin activity is thought to be a primary initiator of ISC transformation. Genetic inactivation of APC is found in ~80% of human patients with CRC, and families harbouring a germline mutation in one APC allele suffer from familial adenomatous polyposis, a disease characterized by the formation of numerous intestinal polyps resulting from stochastic loss of heterozygosity (LOH) at the APC locus, some of which will invariably progress to CRC [14] , [15] , [16] . The role of MSI2 in this process and its potential interaction with the Wnt signalling pathway remains entirely unknown. In this study, we find that MSI2 is overexpressed in human colorectal adenocarcinomas, as well as in early-stage adenomas arising in the APC min/+ mouse model of intestinal tumorigenesis. Using both loss- and gain-of-function approaches we demonstrate that constitutive MSI2 activation is sufficient to phenocopy many histological and molecular aspects of APC loss in the absence of canonical Wnt pathway induction. Transcriptome-wide RNA-binding analysis reveals that MSI2 binds several known intestinal tumor suppressor transcripts, including Pten , a potent tumour suppressor frequently silenced in CRCs. Our findings identify MSI2 as an intestinal oncogene and suggest that MSI2 inhibition may offer a novel point for therapeutic intervention in gastrointestinal (GI) cancers. MSI2 is overexpressed in intestinal cancers To begin understanding the role of MSI2 in CRC, we examined MSI2 expression in human GI cancers, and colorectal adenocarcinomas in particular. Analysis of transcriptome profiles from a number of GI cancers reveals elevated MSI2 in all analysed tumours, including adenocarcinomas of the caecum, colon and rectum ( Supplementary Fig. 1a ). Focusing on colorectal adenocarcinoma, analysis of cancer genome atlas data (TCGA) derived form 314 healthy control individuals and 314 colon adenocarcinomas patient tumours revealed consistent MSI2 overexpression in cancer tissue ( Fig. 1a ). Similarly, analysis of 26 colon adenocarcinoma/adjacent normal tissue pairs from individual patients revealed uniform overexpression of MSI2 in tumours ( Fig. 1b ). Strikingly, MSI2 overexpression was more consistent in these matched samples than that of the well-established colorectal oncogene c-MYC , which was underexpressed in a small fraction of these tumours ( Fig. 1b ). Consistent with the upregulation of MSI2 transcripts, immunohistochemistry analysis of a CRC tissue array confirmed high MSI2 immunoreactivity in all grades of CRC, with an increased MSI2-immunoreactive area correlating with the tumour grade, suggesting that MSI2 activation may be an early event in the ontogeny of cancer ( Fig. 1c and Supplementary Fig. 1b ). We also examined Msi2 expression in intestinal adenomas resulting from LOH of the APC tumour suppressor in the APC min/+ mouse model of intestinal transformation. APC loss occurs in the vast majority of human CRCs, where it is believed to be the initiating oncogenic event. Consistent with our observation in human tumours, adenomas in APC min/+ mice exhibited strong Msi2 immunoreactivity, suggesting a potential role for Msi2 early in intestinal transformation and tumorigenesis ( Fig. 1d ). In order to determine whether Msi2 activation was an immediate early event downstream of APC loss, we deleted APC throughout the epithelium using Villin-CreER [17] and observed a striking upregulation of Msi2 mRNA along with the activation of Wnt target genes ( Axin2, Ascl2 and Lgr5 ) and suppression of differentiation markers Chromogranin-A and Lysozyme characteristic of acute APC loss (ref. 18 ; Fig. 1e ). Thus, Msi2 activation is a direct consequence of APC loss and is characteristic of all grades of colorectal adenocarcinoma. 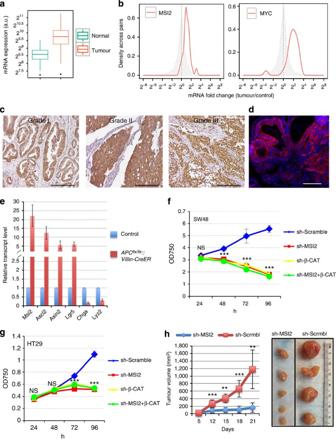Figure 1: MSI2 contributes to human colorectal cancer cell growth. (a) MSI2 mRNA expression levels from RNA-Seq on TCGA (the cancer genome atlas) COAD (colorectal adenocarcinoma) tumour samples (314 solid tissue samples from healthy individuals and 314 tumour samples). Expression values were obtained by TMM normalization of read counts in genes. (b) Fold changes forMSI2(left) andMYC(right) in matched tumour/control RNA-Seq sample pairs from TCGA COAD (total of 26 patients). The distribution ofMSI2/MYCfold changes in tumour/control pairs for 26 individuals is plotted in red (intra-individual comparison). The distribution ofMSI2/MYCfold changes between control/control comparisons for 26 pairs of healthy individuals is plotted in grey (interindividual comparison). (c) MSI2 immunochemistry of graded human colorectal adenocarcinomas (scale bar, 200 μM). (d) Msi2 immunofluorescence showing broad expression in adenomas arising inAPCmin/+mice (scale bar, 200 μM). (e) Expression analysis forMsi2,Wnt target genes (Ascl2, Axin2andLgr5) and differentiation-related genes (ChgaandLyz) in the intestinal epithelium after acute ablation ofAPCinAPCflox/flox::Villin-CreERmice (error bars denotes s.d.,n=3). (f,g) MTT proliferation assays of human colorectal cancer cell lines SW48 (f) and HT29 (g) infected with lentiviral knockdown vectors for MSI2, β-catenin or scramble controls. Error bars indicated s.e.m. from six independent experiments per cell line per condition. ***P<0.0005, Student’st-test. (h) Tumour growth curves of HT29 colon cancer cell xenografts infected with lentivirus expressing scramble control hairpin or sh-MSI2. Error bars denote the s.d. derived from four tumours in each of two mice per group. Representative images of xenograft tumours are shown on the right. **P<0.005, ***P<0.0005, Student’st-test. Figure 1: MSI2 contributes to human colorectal cancer cell growth. ( a ) MSI2 mRNA expression levels from RNA-Seq on TCGA (the cancer genome atlas) COAD (colorectal adenocarcinoma) tumour samples (314 solid tissue samples from healthy individuals and 314 tumour samples). Expression values were obtained by TMM normalization of read counts in genes. ( b ) Fold changes for MSI2 (left) and MYC (right) in matched tumour/control RNA-Seq sample pairs from TCGA COAD (total of 26 patients). The distribution of MSI2/MYC fold changes in tumour/control pairs for 26 individuals is plotted in red (intra-individual comparison). The distribution of MSI2/MYC fold changes between control/control comparisons for 26 pairs of healthy individuals is plotted in grey (interindividual comparison). ( c ) MSI2 immunochemistry of graded human colorectal adenocarcinomas (scale bar, 200 μM). ( d ) Msi2 immunofluorescence showing broad expression in adenomas arising in APC min/+ mice (scale bar, 200 μM). ( e ) Expression analysis for Msi2, Wnt target genes ( Ascl2, Axin2 and Lgr5 ) and differentiation-related genes ( Chga and Lyz ) in the intestinal epithelium after acute ablation of APC in APC flox/flox ::Villin-CreER mice (error bars denotes s.d., n =3). ( f , g ) MTT proliferation assays of human colorectal cancer cell lines SW48 ( f ) and HT29 ( g ) infected with lentiviral knockdown vectors for MSI2, β-catenin or scramble controls. Error bars indicated s.e.m. from six independent experiments per cell line per condition. *** P <0.0005, Student’s t -test. ( h ) Tumour growth curves of HT29 colon cancer cell xenografts infected with lentivirus expressing scramble control hairpin or sh-MSI2. Error bars denote the s.d. derived from four tumours in each of two mice per group. Representative images of xenograft tumours are shown on the right. ** P <0.005, *** P <0.0005, Student’s t -test. Full size image MSI2 promotes cancer cell proliferation and tumour growth To investigate a potential oncogenic role for MSI2 in CRC, we initially performed MSI2 loss-of-function experiments in two human CRC cell lines, SW48 and HT29. Numerous studies have implicated constitutive Wnt pathway activity as a driving force in CRC onset and progression, and these cancers are dependent on the transcription activity of the Wnt effector β-catenin [19] . We therefore knocked down MSI2 alone or in combination with β-catenin and confirmed loss of MSI2 protein using western blot analysis ( Supplementary Fig. 1c ). Surprisingly, MSI2 knockdown completely abrogated growth of SW48 and HT29 cells, and was as potent as loss of β-catenin in growth inhibition ( Fig. 1f,g ). This finding strongly indicates an important role for MSI2 in promoting cancer cell proliferation. We confirmed these in vitro observations by performing xenograft assays on MSI2 knockdown in HT29 cells. Twenty-one days after xenografting, tumour volume was significantly reduced in MSI2 knockdown tumours, with some xenografts exhibiting no growth after transplantation ( Fig. 1h ). MSI2 overexpression largely phenocopies APC loss To gain insight into the potential function of Msi2 in intestinal homeostasis and transformation, we examined Msi2 expression in wild-type mice and found it to be largely restricted to cells of the crypt in the small intestine. This includes crypt base columnar (CBC) stem cells marked by expression of the Wnt co-receptor Lgr5 (ref. 20 ), Paneth cells and the rapidly proliferating cells of the transit-amplifying zone ( Fig. 2a,b , and Supplementary Fig. 2a ). In addition, rare Msi2-positive cells were observed in the differentiated villi, possibly marking enteroendocrine or tuft cells on the basis of frequency and position ( Supplementary Fig. 2a ). We next sought to determine the functional consequences of ectopic MSI2 activity in the intestinal epithelium. We therefore employed a Doxycycline (Dox)-inducible, site-specific, single-copy human MSI2 transgenic mouse model ( TRE-MSI2 ) that we previously utilized to study the oncogenic functions of MSI2 in the haematopoietic system ( Supplementary Fig. 2a ) [4] . Addition of Dox to the drinking water of TRE-MSI2 mice resulted in activation of MSI2 expression throughout the intestinal epithelium within 12 h ( Fig. 2b and Supplementary Fig. 2c ). Strikingly, MSI2 induction resulted in a dramatic expansion of the proliferative zone and an increased frequency of apoptotic cells at the tips of villi, suggesting that cells were being pushed from the crypt to the villus and shed into the lumen at an increased rate ( Fig. 2c,d ). We further observed that differentiated cells of the intestinal epithelium including goblet, enteroendocrine and enterocyte cells were obviously absent in the TRE-MSI2 mice ( Fig. 2e,f and Supplementary Fig. 2d ). However, lysozyme-positive Paneth cells persisted likely due to their long lifespan and stable positioning at the base of the crypt ( Supplementary Fig. 2e ). This block in differentiation resulted in severe dehydration and morbidity within 3–4 days of Dox induction. 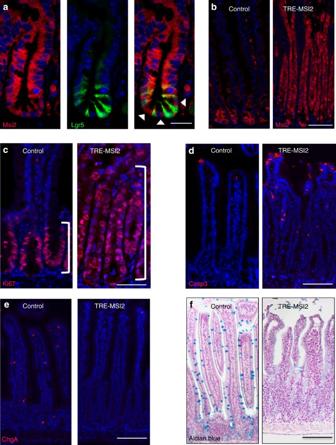Figure 2: MSI2 induction drives intestinal epithelial cell hyperproliferation and blocks differentiation. (a) Immunofluorescence for Msi2 (red) and eGFP (green) in the intestinal crypts ofLgr5-eGFP-IRES-CreERknock-in mice. Msi2 expression is observed in Lgr5+ cells and in adjacent Paneth cells (arrowheads; scale bar, 50 μM). (b–f) Immunofluorescence for MSI2 (b), Ki67 marking proliferating cells (c), cleaved Caspase 3 (Casp3) marking apoptotic cells ind, Chromagranin-A marking enteroendocrine cells (e) and Alcian blue marking Goblet cells (f) in control (M2rtTA) andTRE-MSI2intestines 48 h after 2 mg ml−1Dox induction. Brackets incindicate the crypt-proliferative zone. Scale bars inb–f, 100 μM. Figure 2: MSI2 induction drives intestinal epithelial cell hyperproliferation and blocks differentiation. ( a ) Immunofluorescence for Msi2 (red) and eGFP (green) in the intestinal crypts of Lgr5-eGFP-IRES-CreER knock-in mice. Msi2 expression is observed in Lgr5+ cells and in adjacent Paneth cells (arrowheads; scale bar, 50 μM). ( b – f ) Immunofluorescence for MSI2 ( b ), Ki67 marking proliferating cells ( c ), cleaved Caspase 3 (Casp3) marking apoptotic cells in d , Chromagranin-A marking enteroendocrine cells ( e ) and Alcian blue marking Goblet cells ( f ) in control ( M2rtTA ) and TRE-MSI2 intestines 48 h after 2 mg ml −1 Dox induction. Brackets in c indicate the crypt-proliferative zone. Scale bars in b – f , 100 μM. Full size image To further investigate the effect of MSI2 induction on proliferation and the crypt stem/progenitor cell compartment, we quantified crypt height and crypt fission (frequency of crypts per linear unit) in TRE-MSI2 mice and observed a significant increase in both of these parameters ( Fig. 3a,b ). Interestingly, the increased crypt proliferation, crypt fission, block in differentiation and rapid morbidity in TRE-MSI2 mice are all phenotypes entirely consistent with the consequences downstream of acute APC loss in the intestinal epithelium [18] , [21] . Taken together, these observations suggest that MSI2 induction drives proliferative expansion of an undifferentiated stem/progenitor cell and may act downstream of APC loss to promote intestinal transformation. 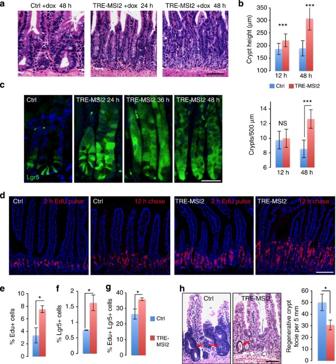Figure 3: MSI2 expression induces crypt fission and expansion of intestinal stem cells. (a) Haematoxylin and eosin staining of control (M2rtTA) andTRE-MSI2small intestine treated with 2 mg ml−1Dox for 24 and 48 h showing expanded crypt height and increased crypt fission (scale bar, 100 μM). (b) Quantification of crypt length (top panel) and crypt fission (lower panel) in control (M2rtTA) andTRE-MSI2intestines at indicated time points after the Dox treatment. Error bars indicate the s.d. derived fromn=3 mice per group per time point. ***P<0.0005, Student’st-test. (c) Immunofluorescence for eGFP in control (Lgr5-eGFP-IRES-CreER::M2rtTA) andTRE-MSI2::Lgr5-eGFP-IRES-CreERintestinal crypts at the indicated time points after Dox induction (scale bar, 50 μM). (d) Histological staining for EdU incorporation 2 or 12 h after an EdU pulse in control (M2rtTA) andTRE-MSI2mice. Images were taken 48 h after initiation of 2 mg ml−1Dox treatment (scale bar, 100 μM). (e) Flow cytometric analysis of EdU incorporation in control (M2rtTA) andTRE-MSI2mice 48 h after 2 mg ml−1Dox induction. Error bars denote s.d. (n=3 mice per group), *P<0.05, Student’st-test. (f,g) Flow cytometric analysis of Lgr5-eGFP+ cell frequency (f) and 2-h-EdU incorporation in Lgr5-eGFP+ cells (g) from control (Lgr5-eGFP-IRES-CreER::M2rtTA) andTRE-MSI2::Lgr5-eGFP-IRES-CreERmice 48 h after 2 mg ml−1Dox treatment. Error bars denote s.d. (n=3 mice per group), *P<0.05, Student’st-test. (h) Histological analysis and quantification of regenerative crypt foci (arrows) in control (Msi2wt/wt::Villin-CreER) orMsi2flox/flox::Villin-CreERmice 3 days after exposure to 12-Gy gamma irradiation (scale bar, 50 μM). Error bars denote s.d. (n=3 mice per group). *P<0.05, Student’st-test. Figure 3: MSI2 expression induces crypt fission and expansion of intestinal stem cells. ( a ) Haematoxylin and eosin staining of control ( M2rtTA ) and TRE-MSI2 small intestine treated with 2 mg ml −1 Dox for 24 and 48 h showing expanded crypt height and increased crypt fission (scale bar, 100 μM). ( b ) Quantification of crypt length (top panel) and crypt fission (lower panel) in control ( M2rtTA ) and TRE-MSI2 intestines at indicated time points after the Dox treatment. Error bars indicate the s.d. derived from n =3 mice per group per time point. *** P <0.0005, Student’s t -test. ( c ) Immunofluorescence for eGFP in control ( Lgr5-eGFP-IRES-CreER::M2rtTA ) and TRE-MSI2 :: Lgr5-eGFP-IRES-CreER intestinal crypts at the indicated time points after Dox induction (scale bar, 50 μM). ( d ) Histological staining for EdU incorporation 2 or 12 h after an EdU pulse in control ( M2rtTA ) and TRE-MSI2 mice. Images were taken 48 h after initiation of 2 mg ml −1 Dox treatment (scale bar, 100 μM). ( e ) Flow cytometric analysis of EdU incorporation in control ( M2rtTA ) and TRE-MSI2 mice 48 h after 2 mg ml −1 Dox induction. Error bars denote s.d. ( n =3 mice per group), * P <0.05, Student’s t -test. ( f , g ) Flow cytometric analysis of Lgr5-eGFP+ cell frequency ( f ) and 2-h-EdU incorporation in Lgr5-eGFP+ cells ( g ) from control ( Lgr5-eGFP-IRES-CreER::M2rtTA ) and TRE-MSI2 :: Lgr5-eGFP-IRES-CreER mice 48 h after 2 mg ml −1 Dox treatment. Error bars denote s.d. ( n =3 mice per group), * P <0.05, Student’s t -test. ( h ) Histological analysis and quantification of regenerative crypt foci (arrows) in control ( Msi2 wt/wt ::Villin-CreER ) or Msi2 flox/flox ::Villin-CreER mice 3 days after exposure to 12-Gy gamma irradiation (scale bar, 50 μM). Error bars denote s.d. ( n =3 mice per group). * P <0.05, Student’s t -test. Full size image APC loss drives intestinal tumorigenesis only when it occurs in an ISC [13] . We therefore sought to assess the effects of MSI2 induction specifically in the ISC compartment. We bred TRE-MSI2 mice to Lgr5-eGFP-IRES-CreER reporter mice that mark CBC stem cells [20] and observed a dramatic expansion of the Lgr5 + zone within the crypts of TRE-MSI2 mice ( Fig. 3c ). This expansion was accompanied by an overall increase in the proliferation rate of intestinal epithelial cells ( Fig. 3d,e ), as well as an increase in the absolute frequency and proliferation rate of Lgr5 + CBCs in TRE-MSI2 mice relative to controls ( Fig. 3f,g ). To test whether the increased apoptotic events at the villus tip in TRE-MSI2 might be a result of increased turnover of the epithelium and more rapid replacement of the differentiated villus compartment with proliferative cells from the crypts, we assessed the migration of ethynyl-2′-deoxyuridine (EdU)-labelled cells after 12 h in the presence of ectopic MSI2 and found that, indeed, proliferative cells in TRE-MSI2 mice migrated higher than their control counterparts ( Fig. 3d ). Taken together, these findings are consistent with a model where MSI2 increases the shedding of differentiated cells and promotes their replacement by undifferentiated cells. To determine whether the effects of MSI2 induction are epithelial cell-autonomous, we cultured crypts from TRE-MSI2::Lgr5-eGFP-IRES-CreER in vitro and observed an increase in crypt budding and Lgr5 + cell expansion, consistent with an epithelial cell-autonomous phenotype ( Supplementary Fig. 3a,b ). Thus, MSI2 induction drives the proliferative expansion of undifferentiated ISCs. This suggests that endogenous Msi2 may play a role in intestinal epithelial proliferation and regeneration. To test this, we first examined regenerative crypt foci 3 days after exposure of wild-type mice to high-dose (12 Gy) gamma irradiation and observed high Msi2 expression in proliferative cells ( Supplementary Fig. 3c ). We next ablated Msi2 expression throughout the intestinal epithelium using Msi2 flox/flox ::Villin-CreER mice [6] and observed that in the absence of Msi2 activity there was a significant decrease in the formation of regenerative crypt foci ( Fig. 3h ), indicating that endogenous Msi2 plays a role in supporting proliferation in the epithelium. MSI2-driven transformation is Msi1-independent Msi2/MSI2 is one of two mammalian orthologues of D. melanogaster Musashi. The second mammalian protein, Msi1/MSI1, is expressed in ISCs and has been implicated as an oncogene in intestinal cancers and elsewhere [11] , [22] , [23] , [24] . We therefore examined Msi1 expression in the TRE-MSI2 intestinal epithelium and observed a striking activation of Msi1 throughout the epithelium in response to MSI2 induction ( Fig. 4a–c ). RNA analysis demonstrates that the activation of Msi1 in response to MSI2 induction occurs at the transcript level, and that the activation is not reciprocal: Msi1 induction in an analogous mouse model ( TRE-Msi1 ) did not result in Msi2 activation ( Fig. 4b ). 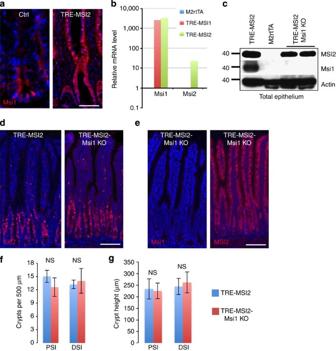Figure 4: Msi1 is dispensable for MSI2-driven intestinal transformation. (a) Immunofluorescence for Msi1 in control (M2rtTA) andTRE-MSI2mice (scale bar, 50 μM). (b) Quantitative RT–PCR for Msi1 and Msi2 in control (M2rtTA),TRE-Msi1 or TRE-MSI2mice treated with 2 mg ml−1Dox for 24 h. Msi1 is induced inTRE-MSI2mice, whereas Msi2 expression is not reciprocally effected byTRE-Msi1induction. (c) Western blot showing Msi1 protein induction on dox treatment ofTRE-MSI2mice. Msi1 induction is prevented inTRE-MSI2::Msi1flox/flox:: VillinCreERmice (TRE-MSI2-Msi1KO) after Tamoxifen-mediated inactivation ofMsi1alleles followed by the Dox treatment. (d) Immunostaining for Ki67 in the intestinal crypts ofTRE-MSI2 and TRE-MSI2::Msi1KOmice (scale bar, 100 μM). (e) Immunofluorescence for Msi1 (left) and Msi2/MSI2 (right) inTRE-MSI2-Msi1KOintestine (scale bar, 100 μM). (f,g) Quantification of crypt fission (f) and crypt height (g) inTRE-MSI2andTRE-MSI2::Msi1KOmice. Error bars indicate s.d. derived from at least 20 fields per slide from each of two mice per condition. PSI/DSI: proximal and distal small intestine. Figure 4: Msi1 is dispensable for MSI2-driven intestinal transformation. ( a ) Immunofluorescence for Msi1 in control ( M2rtTA ) and TRE-MSI2 mice (scale bar, 50 μM). ( b ) Quantitative RT–PCR for Msi1 and Msi2 in control ( M2rtTA ), TRE-Msi1 or TRE-MSI2 mice treated with 2 mg ml −1 Dox for 24 h. Msi1 is induced in TRE-MSI2 mice, whereas Msi2 expression is not reciprocally effected by TRE-Msi1 induction. ( c ) Western blot showing Msi1 protein induction on dox treatment of TRE-MSI2 mice. Msi1 induction is prevented in TRE-MSI2::Msi1 flox/flox :: VillinCreER mice ( TRE-MSI2-Msi1KO ) after Tamoxifen-mediated inactivation of Msi1 alleles followed by the Dox treatment. ( d ) Immunostaining for Ki67 in the intestinal crypts of TRE-MSI2 and TRE-MSI2::Msi1KO mice (scale bar, 100 μM). ( e ) Immunofluorescence for Msi1 (left) and Msi2/MSI2 (right) in TRE-MSI2-Msi1KO intestine (scale bar, 100 μM). ( f , g ) Quantification of crypt fission ( f ) and crypt height ( g ) in TRE-MSI2 and TRE-MSI2::Msi1KO mice. Error bars indicate s.d. derived from at least 20 fields per slide from each of two mice per condition. PSI/DSI: proximal and distal small intestine. Full size image We therefore tested whether the phenotype resulting from MSI2 induction was Msi1-dependent. We generated Msi1 flox/flox ::Villin-CreER mice [25] enabling the deletion of Msi1 within all cells of the intestinal epithelium, and deleted Msi1 , and induced MSI2 with Dox. Msi1 deletion with Villin-CreER resulted in no morphological phenotype during homeostasis consistent with the viability and lack of any overt GI phenotype in germline Msi1 knockout mice [26] . Deletion of Msi1 was confirmed at the protein level ( Fig. 4c,e ). We observed that the phenotype resulting from MSI2 induction was fully penetrant in the absence of Msi1, with increased crypt proliferation and fission, and decreased differentiation being unaffected in TRE-MSI2::Msi1 flox/flox ::Villin-CreER mice ( Fig. 4d–f and Supplementary Fig. 3d ). Thus, Msi1 activity is not required for MSI2-driven transformation of the intestinal epithelium. The oncogenic effects of MSI2 are β-catenin-independent To gain mechanistic insights into the molecular events underlying the effects of MSI2 induction, we analysed transcriptome profiles of intestinal epithelia 24 h after Dox administration to TRE-MSI2 or control ( M2rtTA ) mice, before overt phenotypic changes. MSI2 induction drove rapid and robust changes in the intestinal epithelial transcriptome ( Fig. 5a and Supplementary Table I ). Unbiased gene set enrichment analysis (GSEA) [27] of these changes revealed that the APC-loss gene signature was among the most significantly enriched in the TRE-MSI2 epithelium ( Fig. 5b and Supplementary Fig. 4a,b ). Thus, genes that are activated upon APC loss are also activated upon MSI2 induction, and genes suppressed upon APC loss are similarly suppressed upon MSI2 induction, with a false discovery rate (FDR) approaching zero. 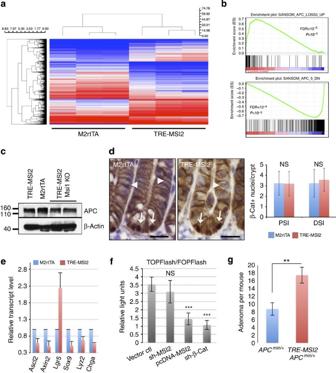Figure 5: MSI2 activation imposes an APC-loss gene signature in the absence of Wnt pathway activation. (a) Hierarchical clustering of transcriptome profiles from the intestinal epithelium of three control (M2rtTA) and threeTRE-MSI2mice 24 h after 2 mg ml−1Dox induction. (b) GSEA of the transcriptome profiles showing a highly significant enrichment of APC loss gene signatures inTRE-MSI2mice. Top panel: genes activated by both APC loss and MSI2 induction; bottom panel: genes suppressed on APC loss and MSI2 induction. FDR: false discover rate. (c) Western blot for APC in lysates of the intestinal epithelium of control (M2rtTA),TRE-MSI2andTRE-MSI2-Msi1KOmice 48 h after 2 mg ml−1Dox induction. (d) Immunohistochemical staining for β-catenin in control (M2rtTA) andTRE-MSI2intestinal crypts 48 h after 2 mg ml−1dox induction, with number of β-catenin+nuclei per crypt section quantified at right (PSI/DSI: proximal and distal small intestine). Error bars indicate the s.d. derived from at least 50 crypts from each mouse (n=3 mice per group, Student’st-test). (e) QRT–PCR analysis of Wnt target gene and differentiation-related gene expression in purified crypts from control (M2rtTA) andTRE-MSI2intestinal crypts 48 h after 2 mg ml−1dox induction. Error bars indicate the s.d.,n=3. (f) β-Catenin/TCF transcriptional reporter activity (TOPFLash) normalized to activity of the reporter with a mutated binding element (FOPFlash) in HEK293 cells upon MSI2 knockdown (sh-MSI2), overexpression (pcDNA-MSI2) or β-catenin knockdown (sh-β-CAT) as a control. Error bars indicate the s.d. (n=4). ***P<0.0005, Student’st-test. (g) Frequency of adenomas inApcmin/+(n=4) andTRE-MSI2::Apcmin/+(n=4) mice treated with low dose Dox (0.1 mg ml−1) in drinking water for 3 weeks. Error bars denote the s.d. **P<0.005, Student’st-test. Figure 5: MSI2 activation imposes an APC-loss gene signature in the absence of Wnt pathway activation. ( a ) Hierarchical clustering of transcriptome profiles from the intestinal epithelium of three control ( M2rtTA ) and three TRE-MSI2 mice 24 h after 2 mg ml −1 Dox induction. ( b ) GSEA of the transcriptome profiles showing a highly significant enrichment of APC loss gene signatures in TRE-MSI2 mice. Top panel: genes activated by both APC loss and MSI2 induction; bottom panel: genes suppressed on APC loss and MSI2 induction. FDR: false discover rate. ( c ) Western blot for APC in lysates of the intestinal epithelium of control ( M2rtTA) , TRE-MSI2 and TRE-MSI2-Msi1KO mice 48 h after 2 mg ml −1 Dox induction. ( d ) Immunohistochemical staining for β-catenin in control ( M2rtTA ) and TRE-MSI2 intestinal crypts 48 h after 2 mg ml −1 dox induction, with number of β-catenin + nuclei per crypt section quantified at right (PSI/DSI: proximal and distal small intestine). Error bars indicate the s.d. derived from at least 50 crypts from each mouse ( n =3 mice per group, Student’s t -test). ( e ) QRT–PCR analysis of Wnt target gene and differentiation-related gene expression in purified crypts from control ( M2rtTA ) and TRE-MSI2 intestinal crypts 48 h after 2 mg ml −1 dox induction. Error bars indicate the s.d., n =3. ( f ) β-Catenin/TCF transcriptional reporter activity (TOPFLash) normalized to activity of the reporter with a mutated binding element (FOPFlash) in HEK293 cells upon MSI2 knockdown (sh-MSI2), overexpression (pcDNA-MSI2) or β-catenin knockdown (sh-β-CAT) as a control. Error bars indicate the s.d. ( n =4). *** P <0.0005, Student’s t -test. ( g ) Frequency of adenomas in Apc min/+ ( n =4) and TRE-MSI2::Apc min/+ ( n =4) mice treated with low dose Dox (0.1 mg ml −1 ) in drinking water for 3 weeks. Error bars denote the s.d. ** P <0.005, Student’s t -test. Full size image In addition to the APC loss gene signature, MSI2 induction significantly enriched gene signatures associated with RNA processing, RAS oncogenic signalling and a common stem cell gene signature, suggesting that MSI2 drives proliferative expansion of an undifferentiated stem/progenitor cell, consistent with the observed increase in Lgr5 + cell frequency and cycling ( Supplementary Fig. 4c ). Further, MSI2 activity strongly suppressed an oxidative phosphorylation expression signature, indicating that a metabolic shift consistent with the Warburg effect may occur in response to MSI2 induction ( Supplementary Fig. 4c ). Given the ability of MSI2 induction to phenocopy many aspects of APC at both the molecular and morphological level, we tested whether MSI2 activation resulted in loss of APC protein, as MSI proteins are known to function as translational repressors [3] . We were unable to detect any decrease in APC upon MSI2 induction ( Fig. 5c and Supplementary Fig. 4d ). Since APC loss is believed to drive transformation of the intestinal epithelium primarily through constitutive activation of the Wnt effector β-catenin and, subsequently, hyperactivation of the canonical Wnt pathway, it was important to address the consequences of MSI2 induction for transcriptionally active (nuclear) β-catenin in TRE-MSI2 crypts. Normally, nuclear β-catenin is limited to the Lgr5 + CBCs and Paneth cells, rapidly disappearing above the +4 position of the crypt ( Fig. 5d ). We observed no change in the pattern or frequency of nuclear β-catenin after MSI2 induction ( Fig. 5d ), or in the expression levels of known direct β-catenin target genes in the transcriptome profiles ( Supplementary Fig. 4e ). We also observed that canonical Wnt target genes such as Ascl2, Axin2, Lgr5 and Sox9 were not among the genes commonly upregulated on APC loss and MSI2 induction in the GSEA ( Supplementary Fig. 4b ). To further explore the effect of MSI2 on activity of the canonical Wnt pathway, we analysed the expression of Wnt target genes Ascl2, Axin2, Lgr5 and Sox9, as well as differentiation markers Lysozyme and Chromogranin-A on MSI2 induction both in crypts in vivo and in organoid cultures. MSI2 had identical effects on the expression of these genes both in vivo and in vitro. Remarkably, not only were Wnt target genes Ascl2, Axin2 and Sox9 not activated, they exhibited suppression on MSI2 induction, providing further evidence that the effects of MSI2 are not mediated through canonical Wnt signalling ( Fig. 5e and Supplementary Fig. 3e ). One exception was Lgr5 , which was activated by MSI2. Differentiation markers Lysozyme and Chromogranin-A were suppressed on MSI2 induction in vivo and in vitro , consistent with the effect of APC loss on differentiation ( Fig. 1e ), and with the effects of MSI2 being epithelial cell-autonomous. Further, in vitro analysis of β-Catenin/TCR reporter activity (TOPFlash) confirmed that MSI2 does not activate canonical Wnt signalling ( Fig. 5f ). We also directly compared the effects of β-Catenin transcriptional activation to MSI2 induction in intestinal organoid cultures from TRE-BcatS33 mice [28] . In these mice, a nondegradable, transcriptionally active β-Catenin is targeted to the identical chromosomal location as MSI2 in the TRE-MSI2 mouse model in the same genetic background, enabling direct comparison of the effects of these two proteins. As expected, induction of β-CateninS33 resulted in the growth of large, spherical, cystic organoids consistent with the known effects of Wnt pathway hyperactivation ( Supplementary Fig. 3f ). In contrast, MSI2 induction resulted in large organoids with prolific crypt budding ( Supplementary Fig. 3f ), consistent with the in vivo phenotype. Consistent with our earlier observation of elevated Msi2 expression in adenomas resulting from LOH in APC min/+ mice and upon acute APC deletion in APC flox/flox mice, these findings support a model in which MSI2 acts downstream of APC loss in a pathway parallel to and independent of β-catenin activation. Thus, MSI2 may cooperate with Wnt/β-catenin signalling to drive tumorigenesis. We therefore crossed TRE-MSI2 mice with APC min/+ mice and administered a low dose of Dox for 3 weeks (0.1 mg ml −1 , or 5% of the standard dose). TRE-MSI2::APC min/+ mice treated with low-dose Dox exhibited an increase in tumour burden resulting from APC LOH, while adjacent tissue that had not undergone LOH remained phenotypically normal ( Fig. 5g and Supplementary Fig. 4f ). This finding provides additional support to the model in which MSI2 promotes tumorigenesis in a pathway parallel to canonical Wnt signalling. Transcriptome-wide MSI2 RNA-binding analysis MSI2 is an RNA-binding protein that, similar to MSI1, harbours two RNA recognition motifs that mediate RNA binding [3] . Binding of RNA targets by MSI1 results in their translational suppression without affecting overall mRNA stability [29] , [30] . Therefore, if we assume that MSI2 (which is highly homologous to MSI1, particularly in the RNA recognition motifs [3] ) acts in a manner similar to MSI1, we expect that the transcriptional changes associated with MSI2 induction are not direct effects of its RNA-binding activity. To identify direct MSI2-binding targets within the intestinal epithelium, we performed crosslinking and immunoprecipitation of Msi2/MSI2-bound RNA in intestinal crypts isolated from wild-type mice and in the TRE-MSI2 -transformed intestinal epithelium, followed by RNase digestion of unprotected RNA and massively parallel sequencing (RNA crosslinking, immunoprecipitation and massively parallel sequencing (CLIP-Seq)). Msi2/MSI2 primarily bound sites in 3′ untranslated regions (UTRs), consistent with the established binding activity of Msi1 (refs 29 , 30 ), and consistent with what we previously observed for MSI2 in haematopoietic cancers [6] ( Fig. 6a ). The vast majority of transcripts bound by Msi2 in wild-type crypts were also bound by ectopic MSI2 (4,387/4,824, or 90%; Fig. 6b ). Conservation analysis of Msi2/MSI2-binding sites revealed that sites in coding sequences and UTRs were significantly conserved relative to flanking sequences; however, this was not true of intronic binding events, suggesting that Msi2/MSI2 binding of introns may represent promiscuous events ( Fig. 6c and Supplementary Fig. 5a ). Limiting analysis specifically to 3′ UTR-bound transcripts reveals a similar overlap between Msi2 targets in wild-type crypts and MSI2-bound targets in the TRE-MSI2 epithelium (91% of Msi2 targets also bound by ectopic MSI2, and 76% of TRE-MSI2 targets also bound by Msi2 in wild-type crypts; Supplementary Fig. 5b ). 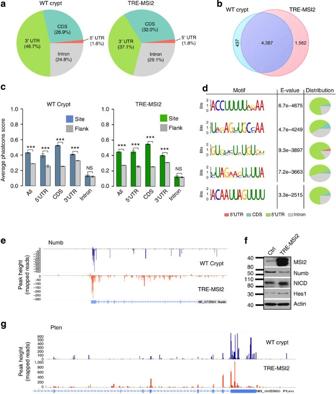Figure 6: Transcriptome-wide MSI2 RNA-binding analysis. (a) CLIP-Seq shows the distribution of Msi2/MSI2 RNA-binding events in wild-type intestinal crypts and theTRE-MSI2epithelium. (b) Venn diagrams show overlap between Msi2/MSI2-bound transcripts in wild-type crypts (left) and theTRE-MSI2epithelium (right) 24 h after 2 mg ml−1Dox induction. (c) PhastCons conservation analysis of Msi2/MSI2 binding quantifying evolutionary conservation of binding sites relative to flanking sequences in all categories with the exception of intronic binding sites (these were not conserved relative to flanking sequences). Error bars represent 95% confidence intervals. ***P<0.0005, two-sample Kolmogorov–Smirnov test. (d) Msi2-binding motif identification and distribution in WT crypts. The previously identified Msi1-binding motif is the final motif pictured. (e) CLIP-Seq track showing Msi2/MSI2 binding to the 3′ UTR of the mRNA encoding Numb. (f) Western blot analysis of Numb, activated Notch (Notch intracellular domain, NICD) and the downstream Notch target geneHes1in control (M2rtTA), and theTRE-MSI2intestinal epithelium. (g) CLIP-Seq track showing Msi2/MSI2 binding to the 3′ UTR of the mRNA-encoding Pten. Figure 6: Transcriptome-wide MSI2 RNA-binding analysis. ( a ) CLIP-Seq shows the distribution of Msi2/MSI2 RNA-binding events in wild-type intestinal crypts and the TRE-MSI2 epithelium. ( b ) Venn diagrams show overlap between Msi2/MSI2-bound transcripts in wild-type crypts (left) and the TRE-MSI2 epithelium (right) 24 h after 2 mg ml −1 Dox induction. ( c ) PhastCons conservation analysis of Msi2/MSI2 binding quantifying evolutionary conservation of binding sites relative to flanking sequences in all categories with the exception of intronic binding sites (these were not conserved relative to flanking sequences). Error bars represent 95% confidence intervals. *** P <0.0005, two-sample Kolmogorov–Smirnov test. ( d ) Msi2-binding motif identification and distribution in WT crypts. The previously identified Msi1-binding motif is the final motif pictured. ( e ) CLIP-Seq track showing Msi2/MSI2 binding to the 3′ UTR of the mRNA encoding Numb. ( f ) Western blot analysis of Numb, activated Notch (Notch intracellular domain, NICD) and the downstream Notch target gene Hes1 in control ( M2rtTA ), and the TRE-MSI2 intestinal epithelium. ( g ) CLIP-Seq track showing Msi2/MSI2 binding to the 3′ UTR of the mRNA-encoding Pten. Full size image Msi2/MSI2 binding was, overall, not selective for the most highly expressed transcripts, and binding did not globally affect overall mRNA levels, as transcripts newly bound on MSI2 induction in the TRE-MSI2 epithelium exhibited no change in mRNA levels ( Supplementary Fig. 5c–e ). This is consistent with MSI2 RNA interaction promoting neither mRNA degradation nor stabilization. Binding motif analysis for Msi2 in wildtype (WT) crypts revealed that Msi2 bound a number of U-rich motifs, and the previously published Msi1-binding motif [(G/A)U( n )AGU ( n =1–3)] (ref. 29 ), while not among the most significant, was still highly enriched and significant in the data ( Fig. 6d ). Electrophoretic mobility shift assays confirmed the interaction of recombinant human MSI2 with the dominant 3′ UTR motif 5′-ACCUUUUUAGAA-3′ ( Supplementary Fig. 5f ). Global analysis of Msi2 RNA-binding targets revealed an enrichment in transcripts encoding proteins involved in protein localization and transport, ribosome biology and nucleotide/ribonucleotide binding, consistent with what was observed previously for MSI2 in haematopoietic cancers [6] ( Supplementary Fig. 6a ). Interestingly, mRNA targets involved in neurodegenerative diseases including Parkinson’s, Alzheimer’s and Huntington’s were also significantly enriched, possibly reflecting a role for MSI2 in these disorders ( Supplementary Fig. 6a ). We next examined the binding of Msi2 to transcripts that have previously been identified as Msi1-binding targets in vitro , including Cdkn1a (encoding p21) and Numb [29] , [30] . Msi2/MSI2 bound both Cdkn1a and Numb mRNAs in their 3′ UTRs ( Fig. 6e and Supplementary Fig. 6b ). Interestingly, MSI2 induction had only modest effects reducing the Numb protein and activating Notch signalling, and no enrichment for a Notch expression signature was observed in our transcriptome profiles, indicating that Notch activation is not a major consequence of MSI2 induction. These data validate our CLIP-Seq approach and indicate that Msi2 has an RNA-binding activity similar to the second mammalian Musashi family member, Msi1. Given the observed binding of MSI2 to the transcripts encoding the tumour suppressors p21 and Numb, we examined the CLIP data set for other interactions between MSI2 and tumour suppressors. Remarkably, MSI2 bound several well-established intestinal tumour suppressions including Lrig1 (ref. 31 ), Bmpr1a (ref. 32 ) and Pten [33] , [34] ( Fig. 6f and Supplementary Fig. 6b ). Interestingly, PTEN protein is lost in many CRCs; however, the PTEN gene is rarely the target of genetic inactivation [35] . Thus, it is tempting to speculate that binding of PTEN mRNA by MSI2 may account for the loss of the PTEN protein in PTEN- wild-type cancers. MSI2 inhibits Pten and activates the mTORC1 pathway PTEN is a well-known tumour suppressor in CRC and has been implicated in the regulation of ISCs [33] . Deletion of Pten in the context of APC deficiency accelerates adenoma formation and activates the PDK–AKT–mTORC1 pathway [33] , [34] , [36] . To investigate the possibility that MSI2-mediated transformation of the intestinal epithelium is a result of Pten inhibition, we examined Pten protein levels and observed a reduction on TRE-MSI2 induction ( Fig. 7b ). Pten is a phosphatase that dephosphorylates phosphatidylinositol (3,4,5)-triphosphate (PIP3), converting it to PIP2. Loss of Pten thus blocks the conversion of PIP3 to PIP2, leading to an accumulation of PIP3. Analysis of PIP3 in both total intestinal epithelial cells and specifically in Lgr5 + CBC stem cells reveals an increase in PIP3-positive cells after TRE-MSI2 induction, consistent with an inhibition of Pten activity ( Fig. 7b ). 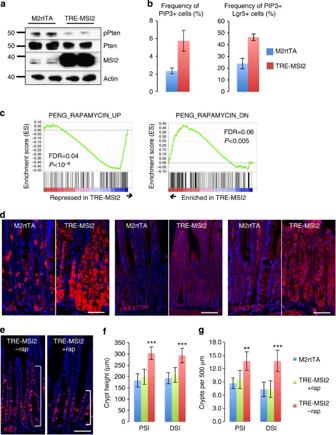Figure 7: Activation of the Pten–AKT–mTORC1 axis is necessary for MSI2 transformation of the intestinal epithelium. (a) Western blotting showing reduction of the Pten protein inTRE-MSI2crypts versus controls (M2rtTA) 48 h after 2 mg ml−1Dox induction. (b) Flow cytometric quantification of PIP3+cell frequency in total intestinal epithelial cells (left) andLgr5-eGFP+crypt base columnar stem cells in (right) between control (M2rtTA) andTRE-MSI2mice 48 h after Dox induction (n=3 mice per group), error bars indicate the s.d. (c) GSEA demonstrating an inverse correlation between theTRE-MSI2transcriptome and Rapamycin-regulated genes. Genes upregulated by the Rapamycin treatment are suppressed by MSI2 (left), and genes suppressed by the Rapamycin treatment are upregulated by MSI2 induction. (d) Immunofluorescence for pS6, p-AKT (T308) and p-AKT (s473) showing activation of the AKT/mTORC1 signalling axis inTRE-MSI2mice (scale bar, 50 μM). (e) Immunofluorescence staining for Ki67 in Dox-inducedTRE-MSI2mice treated with or without Rapamycin (scale bar, 50 μM). (f,g) Qualification of crypt height infand crypt frequency ingin control (M2rtTA),TRE-MSI2and Rapamycin-treatedTRE-MSI2mice. Error bars denote s.d. Crypt height was measured based on 40 crypts in each of three independent pairs of mice. Crypt frequency was scored in 20 randomly selected areas in proximal and distal intestine (PSI and DSI, respectively) in each of three independent pairs of mice. **P<0.005, ***P<0.0005. Figure 7: Activation of the Pten–AKT–mTORC1 axis is necessary for MSI2 transformation of the intestinal epithelium. ( a ) Western blotting showing reduction of the Pten protein in TRE-MSI2 crypts versus controls ( M2rtTA ) 48 h after 2 mg ml −1 Dox induction. ( b ) Flow cytometric quantification of PIP3 + cell frequency in total intestinal epithelial cells (left) and Lgr5-eGFP+ crypt base columnar stem cells in (right) between control ( M2rtTA ) and TRE-MSI2 mice 48 h after Dox induction ( n =3 mice per group), error bars indicate the s.d. ( c ) GSEA demonstrating an inverse correlation between the TRE-MSI2 transcriptome and Rapamycin-regulated genes. Genes upregulated by the Rapamycin treatment are suppressed by MSI2 (left), and genes suppressed by the Rapamycin treatment are upregulated by MSI2 induction. ( d ) Immunofluorescence for pS6, p-AKT (T308) and p-AKT (s473) showing activation of the AKT/mTORC1 signalling axis in TRE-MSI2 mice (scale bar, 50 μM). ( e ) Immunofluorescence staining for Ki67 in Dox-induced TRE-MSI2 mice treated with or without Rapamycin (scale bar, 50 μM). ( f , g ) Qualification of crypt height in f and crypt frequency in g in control ( M2rtTA ), TRE-MSI2 and Rapamycin-treated TRE-MSI2 mice. Error bars denote s.d. Crypt height was measured based on 40 crypts in each of three independent pairs of mice. Crypt frequency was scored in 20 randomly selected areas in proximal and distal intestine (PSI and DSI, respectively) in each of three independent pairs of mice. ** P <0.005, *** P <0.0005. Full size image Accumulating PIP3 binds to PDK1, in turn activating the AKT–mTorc1 pathway [37] . Consistent with Pten suppression and mTORC1 activation downstream of MSI2 induction, GSEA revealed an inverse correlation between the TRE-MSI2 gene signature and the Rapamycin gene signature ( Fig. 7c ). Rapamycin is a potent inhibitor of the mTORC1 complex, and thus these findings indicate that the mTORC1 complex is being activated by MSI2 induction. We further examined activity of the pathway downstream of Pten and observed increased phosphorylation of AKT (Phospo-AKT (T308) and Phospo-AKT (S473) , Fig. 7d ), as well as increased mTORC1 activity, assessed by phosphorylation of S6 by S6 kinase and phosphorylation of 4EBP1 ( Fig. 7d and Supplementary Fig. 7a ). Ultimately, we asked whether MSI2-mediated mTORC1 activation functionally contributes to intestinal transformation in TRE-MSI2 mice. Since it is well established that mTORC1 activity is dispensable for intestinal homeostasis [38] , [39] , we blocked mTORC1 signalling in TRE-MSI2 mice with Rapamycin for 2 days before Dox induction of MSI2 for 48 h. Phosphorylation of S6 was markedly reduced in Rapamycin-treated TRE-MSI2 mice ( Supplementary Fig. 7b ), confirming that mTORC1 activity was effectively inhibited. Strikingly, we found that the expanded proliferative zone within the crypts marked by Ki67 in TRE-MSI2 mice was fully rescued by the Rapamycin treatment ( Fig. 7e,f ). Furthermore, we observed that the increase in crypt density/crypt fission was also rescued in the Rapamycin-treated TRE-MSI2 mice, demonstrating that activation of mTORC1 functionally contributes the increased crypt fission and hyperplasia observed in TRE-MSI2 mice ( Fig. 7g ). In summary, these findings demonstrate that MSI2 is a potent oncogene capable of recapitulating phenotypes resulting from APC loss through the activation of mTORC1 in an unappreciated, Wnt-independent oncogenic pathway. Here we identify MSI2 as a potent oncogene in CRC. The current dogma of CRC initiation suggests that loss of the APC tumour suppressor results in the failure to degrade β-catenin, consequently resulting in constitutive activation of the Wnt signalling pathway. This process is believed to result in tumorigenesis only when it occurs in ISCs, as genetic ablation of APC in other cell types of the intestine does not initiate tumorigenesis [13] . In the current study we observe high levels of MSI2 in primary human CRCs, along with Msi2 induction upon the loss of APC in mouse models. Further, we observe that loss of MSI2 abrogates growth of CRC cells (both APC-wild-type and APC-negative), where its loss is as effective as loss of β-catenin in inhibiting CRC cell growth. These findings, coupled with our previous findings in acute and chronic myelogenous leukaemias [4] , indicate that MSI2 is upregulated in a number of cancers (possibly through a variety of mechanisms, as elevated MSI2 levels are found in cancers with distinct underlying genetic mutations), and that these cancers become dependent on oncogenic MSI2 activity. In the current study we sought to model the consequences of MSI2 induction on the intestinal epithelium. Using a single-copy, drug-inducible MSI2 transgenic mouse model we are able to rapidly and robustly induce MSI2 activity throughout the intestinal epithelium. Strikingly, MSI2 activity alone was sufficient to phenocopy many aspects of APC loss in the intestinal epithelium (the exception being Paneth cell mislocalization), resulting in a dramatic expansion of the crypt-proliferative zone, a block in differentiation and an increase in crypt fission [18] . This phenotype was also reflected at the molecular level, with unbiased GSEA of the MSI2-expressing epithelium identifying the APC loss gene signature among the most significantly enriched. Given the dogma that APC loss drives intestinal cancer through constitutive Wnt pathway activation, we examined whether Wnt hyperactivation could contribute to the TRE-MSI2 phenotype and, surprisingly, found no evidence of Wnt pathway activation, either at the level of APC loss, nuclear β-catenin localization or β-catenin target gene activity. This result prompts a reassessment of the dogma that constitutive β-catenin activity is the sole oncogenic consequence of APC loss, a notion that is supported by recent evidence that constitutive β-catenin activation is not sufficient to recapitulate many phenotypes associated with APC loss [28] , [40] . Taken together, our findings suggest that MSI2 activation represents an oncogenic pathway downstream of APC loss and parallel to β-catenin activation. This concept runs contrary to recent in vitro reports that the second mammalian MSI family member, MSI1, activates canonical Wnt signalling [24] , [41] , [42] , possibly reflecting differences between the in vivo setting used in the current study and the in vitro approaches taken in published studies, as well as tissue-specific differences, as only one of these studies examined CRC cells in vitro [41] . Given the evidence for functional redundancy between the two mammalian MSI proteins [26] , and that MSI1 appears to have an oncogenic role in CRC cell lines [23] , we also examined Msi1 expression in our TRE-MSI2 mouse model and observed a striking induction of Msi1 at the mRNA level; however we conclude, through Msi1 loss-of-function studies, that the oncogenic properties of MSI2 are not dependent on Msi1, although this certainly does not rule out an oncogenic role for Msi1/MSI1 independently of Msi2/MSI2. The co-expression of both Msi proteins in stem cells of the intestinal crypt (this study and ref. 10 ), the lack of any major intestinal phenotype described in either germline Msi1 knockout mice [26] and our conditional Msi1 flox/flox ::VillinCreER mice (this study), along with the aforementioned functional redundancy of Msi proteins [26] raises the intriguing possibility that Msi proteins act redundantly to maintain stem cell self-renewal in the ISC compartment, as we have previously observed for Msi2 in HSCs [6] . It will be important to address this possibility in future studies utilizing dual- Msi conditional knockout mice. Transcriptome-wide RNA-binding analysis of endogenous Msi2 in intestinal crypts, ectopic MSI2 in the intestinal epithelium and of MSI2 in human leukaemic cell lines offers insight into the tissue-specific versus common functions of MSI2 in these tissues. In the intestinal transcriptome analysed in this study and the leukaemic transcriptome analysed in ref. 6 , MSI2 bound to transcripts involved in RNA biogenesis and metabolism, suggesting that MSI regulation of these fundamental biological processes may be conserved across tissues. Pathway analysis in haematopoietic tissues indicates that MSI2 primarily acts to modulate TGF-β signalling, whereas in the intestinal epithelium, the Pten–AKT–mTORC1 axis was identified as being a major target of MSI2 activity, indicating that MSI2 may have cell-type-specific functions (although the mTOR pathway was also identified as an MSI2 target in the haematopoietic system, it appears not to be as dramatically affected as in the intestinal epithelium). Conceptually, this phenomenon is not unexpected as RNA-binding protein activity must, by definition, be restricted to the repertoire of transcripts expressed in a particular cell type. This is in contrast to transcription factors, whose DNA targets are identical in all cell types, epigenetic-regulated accessibility and cofactor binding notwithstanding. Thus, MSI2 and other RNA-binding proteins might serve as hubs of signal integration by acting on mRNAs in the cytoplasm, with the possibility of cell-type-specific function depending on the mRNA repertoire available for binding in any given cell type. In the current study, we identify the Pten–AKT–mTORC1 axis as a major MSI2 target with functional relevance to the observed phenotype; however, we note that MSI2 binds numerous additional tumour suppressors with known roles in CRC, including Cdkn1a, Lrig1, Bmpr1a and Numb. At least two of these targets (Bmpr1a and Lrig1, in addition to Pten) are also known repressors of mTorc1, and thus the effects of MSI2 on mTorc1 activity may be the result of pleiotropic inhibition of these tumour suppressors. While such pleiotropic inactivation of tumour suppressors may make MSI2 a potent oncogene, it also represents an attractive point for therapeutic intervention. In principle, MSI2 inhibition may allow for the concerted re-activation of this cadre of colorectal tumour suppressors. Thus, the viability of MSI2 as a drug target will be of great interest moving forward in the fight against CRC, and likely a variety of other cancers. Mouse strains All procedures involving mice were reviewed and approved by the Institutional Animal Care and Use Committee of the University of Pennsylvania (Animal Welfare Assurance Reference Number no. A3079-01, approved protocol no. 803415 granted to Dr Lengner) and were in accordance with the guidelines set forth in the Guide for the Care and Use of Laboratory Animals of the National Research Council of the National Institutes of Health. The generation of TRE-MSI2 mice is described in ref. 4 . Briefly, the human MSI2 cDNA (open biosystems clone IDno. 5942 Accession CV027635) under control of the tetracycline operator with a minimal CMV promoter was targeted to safe-haven chromatin downstream of the Collagen1a1 locus in KH2 embryonic stem cells also harbouring the modified reverse tetracycline transactivator (M2rtTA) targeted to and under transcriptional control of the ROSA26 locus [43] . Lgr5-eGFP-CreER mice were obtained from Jackson Laboratories (stock no. 008875). Conditional loss-of-function Msi1 flox/flox mice will be described in detail elsewhere. Briefly, the two exons, including the transcriptional start site of Msi1 , were targeted with flanking LoxP sites resulting in the 2lox, or floxed locus. Deletion of this region results in the loss of the transcriptional start site and a frameshift in the Msi1-coding sequence. Proper recombination at both the 5′ and 3′ ends of the arms of homology was confirmed by Southern blotting. Mice generated from 2lox ES cells were bred to homozygosity and crossed with Villin-CreER mice [17] . Msi1 was conditionally deleted by administration of five consecutive doses of Tamoxifen (50 mg kg −1 ) in corn oil (Sigma), and loss of Msi1 /Msi1 was confirmed by Southern blotting, quantitative reverse transcription–PCR (qRT–PCR) and immunostaining. Dox induction of MSI2 in TRE-MSI2::Msi1 flox/flox ::VillinCreER mice was initiated 5 days after the final dose of Tamoxifen. TRE-B-CatS33 (ref. 28 ) mice were a kind gift of Dr Konrad Hochedlinger. For ablation of APC, APC flox/flox mice [44] were crossed with Villin-CreER mice and APC was deleted with four consecutive daily doses of Tamoxifen (50 mg kg −1 ) in corn oil (Sigma). Epithelial RNA was isolated 5 days after the initial Tamoxifen dose and processed for qRT–PCR as described below. The generation of Msi2 flox/flox mice is described in ref. 6 . Gamma irradiation after Msi2 deletion in Msi2 flox/flox ::Villin-CreER mice was performed on at least four mice in each of knockout and control groups, treated with five consecutive doses of Tamoxifen (50 mg kg −1 ) in corn oil (Sigma) followed by 5 days of recovery and exposure to 12 Gy whole-body γ-irradiation. Controls and experimental mice were sex-matched littermates. Intestines were washed with PBS, fixed in 4% paraformaldehyde, paraffin-embedded and sectioned. Surviving crypts were defined as 10 or more adjacent chromophilic cells and a lumen in haematoxylin and eosin-stained sections from the intestinal epithelium. Dox induction and isolation of the intestinal epithelium For Dox induction experiments of control ( M2rtTA +/+ ) and TRE-MSI2 +/− ::M2rtTA +/+ mice, 2 mg ml −1 Dox (Doxycycline hyclate, Sigma) was added to the drinking water along with 1% w/v sucrose of mice 8–10 weeks of age. All experiments except tumour formation in TRE-MSI2::APC min/+ mice utilized the 2-mg ml −1 Dox dosage in mice homozygous for M2rtTA and heterozygous for the TRE-MSI2 allele. Most experiments were conducted after 48 h of exposure to Dox-containing drinking water, with the exception of transcriptome profiling, which was carried out 24 h after the initiation of Dox treatment. For APC min/+ experiments, TRE-MSI2 +/− ::APC min/+ ::M2rtTA +/− or APC min/+ ::M2rtTA +/− (in these experiments the M2rtTA was heterozygous to reduce MSI2 dosage) were administered 0.1 mg ml −1 of Dox in the drinking water for 3 weeks starting at 2 months of age while being fed low-protein/high-fat diet (Research Diets, D12079B). For isolation of whole-intestinal epithelial cells, the mouse intestine was cut longitudinally and washed two to three times with ice-cold Dulbecco's phosphate buffered saline (DPBS), then cut into small pieces (3–7 mm long) and incubated for 1 h at 4 °C in DPBS containing 2 mM EDTA and 0.2 mM dithiothreitol on a rotating platform, and collecting suspended cells after gentle vortexing. For isolation of intestinal crypts, mouse small intestine was washed with DPBS as above. The villi were scraped using a hemocytometer coverslip. The crypts were released by incubation for 30 min at 4 °C in DPBS containing 2 mM EDTA and gentle vortexing. Isolated crypts were counted and pelleted as described in ref. 45 . Flow cytometry The intestine was cut open longitudinally and incubated with 5 mM EDTA-HBSS solution at 4 °C for 30 min. Single cell suspension was generated with Dispase (BD Biosciences, San Jose, CA). Flow cytometry analysis was performed with BD LSR Fortessa cell analyzer (BD Biosciences). 4',6-diamidino-2-phenylindole (DAPI)-negative cells were selected, and then gated for single cell based on Forward-scatter height versus forward-scatter width and side-scatter height versus side-scatter width profiles. The size of the nozzle for all sorting is 100 μm (20 psi). Lgr5+ stem cells were quantified by flow cytometry in TRE-MSI2::Lgr5-eGFP-IRES-CreER and M2rtTA::Lgr5-eGFP-IRES-CreER control mice after 48 h of the Dox treatment. EdU labelling and flow cytometry TRE-MSI2::Lgr5-eGFP-IRES-CreER and M2rtTA::Lgr5-eGFP-IRES-CreER control mice were treated with 2 mg ml −1 Dox (Sigma) and were injected with 0.15 mg of 5-EdU (Life Technologies) 2 or 12 h before killing and intestinal isolation. The intestine was cut open longitudinally and washed twice with ice-cold PBS. The intestine was incubated with 30 mM EDTA (EDTA, Sigma) and 1.5 mM DTT (Sigma) in HBSS at 4 °C for 20 min. Then, it was moved to 30 mM EDTA in HBSS at 37 °C for 10 min and dissociated by pipetting vigorously. Single-cell suspension was generated with 0.8 mg ml −1 Dispase (GIBCO) [46] . Cells were fixed with Click-iT fixative (Life Technologies) for 15 min at room temperature and stained with FITC-anti-GFP (fluorescein isothiocyanate-anti-green fluorescent protein; Abcam) for 30 min on ice and washed twice with Click-iT permeabilization and wash reagent. For Click-it labelling, cells were incubated with CuSO 4 and Alexa fluor 647 azide dye as per the user manual and cells were analysed using flow cytometry. Flow cytometry was performed on an LSR Fortessa, and the Flowjo software was used for data analysis. PIP3 flow cytometry Intestinal epithelial cells were suspended in PBS containing 1 μl ml −1 of fixable viability dye eFluor 450 (Affymetrix ebioscience). Cells were incubated on ice for 30 min and were washed two times with PBS. Then, cells were fixed and permeabilized using Cytofix/Cytoperm solution (BD PharMingen), stained with FITC-anti-GFP (Abcam) and biotinylated anti-PIP3 (Echelon Inc.) for 30 min on ice and washed twice. They were incubated with Streptavidin-APC(Biolegend) for 30 min on ice and washed twice. Flow cytometry was performed on an LSR Fortessa, and the Flowjo software was used for data analysis. Administration of Rapamycin Rapamycin (LC Laboratories) was administered by daily intraperitoneal injection (4 mg per kg of body weight) for 5 days. It was reconstituted in absolute ethanol at 10 mg ml −1 and diluted in 5% Tween-80 (Sigma) and 5% PEG-400 (Hampton Research) before injection. The final volume of all injections was 200 μl. Dox was administered to TRE-MSI2 mice as above for 48 h after the third dose of Rapamycin. Crypt organoid culture and qRT–PCR from the intestinal epithelium and organoids Crypt culture was performed as previously described in ref. 45 . After intestinal crypt isolation, a total of 500 crypts were mixed with 50 μl of Matrigel (BD Bioscience) and plated in 24-well plates. After polymerization of Matrigel, 500 μl of crypt culture medium (Advanced DMEM/F12 containing 50 ng ml −1 EGF (Invitrogen), 1 μg ml −1 R-spondin (Wistar Institute protein production facility), 100 ng ml −1 Noggin (Peprotech) and 3 μM GSK-3 inhibitor CHIR99021 (Stemgent) was added. After 2-day culture at 37-°C incubator, the organoids were treated with 2 μg ml −1 Dox and harvested for qRT–PCR analysis 72 h later. RNA was isolated from organoids, crypts or total epithelium, using QIAGEN RNeasy mini plus kits. Total RNA (1 μg) was used for cDNA synthesis. Primers used in qRT–PCR are as follows: Histological analyses Intestines were washed with DPBS, fixed in 10% formalin, paraffin-embedded and sectioned. Haematoxylin, eosin, Alcian blue and alkaline phosphatase staining were performed in the Morphology Core of the Penn Center for Molecular Studies in Digestive and Liver Diseases. For immunohistochemistry staining, antigen retrieval was performed by heating slides in 0.01 M citrate buffer (pH 6) with a pressure cooker. The sections were then immunostained by the ABC peroxidase method (Vector Laboratories) with diaminobenzidine as the enzyme substrate and haematoxylin as a counterstain. For detection of nuclear β-catenin, antibody clone 15B8 (Sigma; 1:1,000) was used in combination with the MOM kit (Vector Laboratories). For immunofluorescence staining, paraffin sections were pretreated in 0.01 M citrate buffer (pH 6) with a pressure cooker, and incubated in primary antibodies, then incubated with Cy2- or Cy3-conjugated fluorescent secondary antibodies (Jackson Laboratory) and counterstained with DAPI in mounting media (Vector Laboratories). For amplification of signal from Msi1 and Msi2, we used a Biotin-Streptavidin system. The following antibodies were used: Ki67 (1:1,250, Leica), Msi1 (1:400, MBL), Msi2 (1:200, Novus Biologicals), Lysozyme (1:50, Santa Cruz), Chromogramin A (1:1,000, Abcam), GFP (1:200, Abcam), pS6 (1:200; Cell Signaling), p-AKT (T308; 1:200; Cell Signaling), p-AKT (S473; 1:200; Cell Signaling), p-4EBP1 (T37/46; 1:200; Cell Signaling). CLIP-Seq Clip libraries were made as previously described in ref. 47 with minor modification. Total intestinal epithelial cells from TRE-MSI2 mice treated with Dox for 24 h were isolated as above, and wild-type intestinal crypts were isolated as above. For crosslinking, cell suspension was exposed to two pulses of 265 nm UV light at 400 mJ cm −2 in a Stratalinker (Model 2400, Stratagene). Epithelial cells were then lysed using PXL buffer (PBS, 01% SDS, 0.5% deoxycholate, 0.5% NP-40, plus protease inhibitor and RNAsin). The lysates were sequentially treated with DNaseI and RNase, and spin in ultramicrocentrifuge at 40,000 g for 20 min. The supernatant was added to protein A Dynabeads (Dynal, 100.02) conjugated with MSI2 antibody (EMD Millipore 03-115) and incubated for 4 h at 4 °C. The 32P-γ-ATP-labelled 3′ RNA (RL-3) linker was ligated to the RNA fragment on beads overnight at 16 °C. The beads were re-suspended in 30 μl of Novex loading buffer (without reducing agent), and separated with Novex NuPAGE 10% Bis-Tris gel and transferred to S&S BA-85 nitrocellulose membrane. After overnight exposure, an ~50-KDa band was visualized and the corresponding membrane was cut into small pieces. The RNA was released by proteinase K digestion and isolated using RNA phenol and CHCl3 solution. The 5′ RNA (RL-5) linker was ligated into the RNA fragments. The RNA was transcribed into complementary DNA using RT–PCR and amplified using Re-PCR with Solexa fusion primers. The CLIP library underwent single-end sequencing on an Illumina hiSeq2000 at the University of Pennsylvania Functional Genomics Core. RL-3: 5′-OHGUGUCAGUCACUUCCAGCGG-3′—puromycin; RL-5: 5′-OHAGGGAGGACGAUGCGG-3′-OH. Adapter sequences were removed from the 3′ end using cutadapt ( http://journal.embnet.org/index.php/embnetjournal/article/view/200 ) with options '-a GTGTCAGTCACTTCCAGCG -e 0.06 -O 6 -m 12′. Reads were then mapped to the mouse (mm9) transcriptome and genome using Tophat [48] with options ‘--read-mismatches 1 --read-gap-length 1 --read-edit-dist 1 --max-multihits 100 --b2-very-sensitive --transcriptome-max-hits 100 --no-coverage-search --no-novel-juncs’. Peaks were called using Piranha [49] with a window size of 200 bp. Motifs were identified using the MEME software suite [50] . Transcriptome profiling Total RNA was isolated from total mouse small intestinal epithelial cells from three M2rtTA and three TRE-MSI2 mice administered Dox for 24 h in the drinking water (as above) using TRIzol Reagent (Life Technologies) according to the manufacturer’s instructions. Total RNA was DNAse-treated with an RNAse-free DNAse kit (Zymo Research). Purified RNA was submitted to the University of Pennsylvania Molecular Profiling Core, where samples were labelled and hybridized to Affymetrix Mouse Gene 1.0ST arrays. Microarray data were analysed using the Partek Genomics SuiteTM software. Following RMA background subtraction and normalization, a one-way analysis of variance (ANOVA) between controls (M2rtTA) and MSI2-induced (TRE-MSI2) was run to compute P values of significance and F-statistic for each probe set. q value, a measure of FDR, was computed within the Significance Analysis of Microarrays software for each probe set by running an unpaired t -test. The FDR values were integrated with the one-way ANOVA results. Genes that were significant at FDR cutoff of 5% and changed at least twofold in either direction in the MSI2 induction group when compared with the control group were selected as the set of differentially expressed genes. This set of 836 unique genes and 6 samples were subjected to agglomerative hierarchical clustering analysis. Log2 intensities were median-centred across samples. Euclidean distance was used as the dissimilarity metric and average linkage method as clustering strategy. Results were visualized as intensity heatmap ( Fig. 5a ). For analysis of direct β-catenin target gene expression in Fig. 5f , genes with published evidence for direct regulation by β-catenin demonstrated by chromatin immunoprecipitation were selected. These genes include Edn1, Fra- 1 (Fosl1), c-Myc, Met, c-Jun, Pinx1, Tcf4, Egfr, Klf5, Cyclin D ( Ccnd1 ), Mycbp, Mmp7, Cdkn2a, Vegfa, SNAI1, Fgf18, Gja1 ( connexin-43 ), Axin2, Claudin1, Runx2, Lef1, Bglap, ENPP2, Nrcam, DLK1, Vcan, Fgf4, Fn1, Tcf1 , (Hnf1a), Lgr5, Ppard, Sp5, Ovol1, Id2, L1CAM, Cdh1 ( E-cadherin ) , Fst, Tnfrsf19, Neurod1, Ctla4, Wisp1, Fzd7, Mitf, Pou3f2, Gbx2, Nkx2-2, Neurog1, Eda, T, Pitx2, Btrc, Cdx1, Birc5 ( survivin ), Pkd1, Pml, and Lect2 ( chemotaxin2 ). Oncomine and TCGA Using Oncomine analysis, the MSI2 expression level was analysed in the Kaiser colon database. The database includes full transcriptome profiles of 105 samples: Control (5); caecum adenocarcinoma (17); colon adenocarcinoma (41); colon mucinous adenocarcinoma (13); colon signet ring cell adenocarcinoma (2); colon small cell carcinoma (2); rectal adenocarinoma (8); rectal mucinous adenocarcinoma (4); rectal signet ring cell adenocarcinoma (1); rectosigmoid adenocarcinoma (10); and rectosigmoid mucinous adenocarcinoma (2; ref. 51 ). For TCGA analysis, mRNA expression levels from RNA-Seq on TCGA COAD tumour samples (314 solid tissue samples from healthy individuals and 314 tumour samples) were analyzed. Expression values were obtained by trimmed mean of M-values (TIMM) normalization of read counts in genes. Fold changes for MSI2 in matched tumour/control RNA-Seq sample pairs from TCGA COAD were calculated (total of 26 patients.) Distribution of MSI2 fold changes in tumour/control pairs for 26 individuals plotted are in red (intraindividual comparison). Distribution of MSI2 fold changes between control/control comparisons for 26 distinct individuals plotted in grey (interindividual comparison). Cell proliferation assays SW48 (ATCC stock number CCL-231) and HT29 (ATCC stock number HTB-38) were seeded in 96-well plates at a density of 1,500 and 2,000 cell and cultured in DMEM supplemented with 10% FBS, 1% sodium pyruvate, 1% penicillin/streptomycin and 1% L-glutamine 24 h before infection. For infection, the medium was removed, and cells were gently washed with PBS. Viral supernatant (100 μl) containing pSICO-eGFP-shScramble, -sh-MSI2, -sh-BCAT and -sh-MSI2 & -sh-BCAT. Cell proliferation assays were performed using MTT (3-[4, 5-dimethylthiazol-2-yl]-2, 5-diphenyltetrazolium bromide) assays. Absorbance was measured at 570 nm. All data ware expressed as a mean from at least three independent biological experiments with n =4 per condition per experiment. Xenograft assays Six-week-old female nude mice were obtained from the Stem Cell and Xenograft Core at UPENN. Stably infected CRC cells were trypsinized and suspended in PBS. A total volume of 0.2 ml containing 2–5 × 10 6 cells and 25% volume MatriGEL was injected subcutaneously into the mouse flank. Tumour size was measured using a Vernier caliper. Tumour volumes were calculated using the formula V =1/2 ( L × W 2 ), where L is length (longest dimension) and W is width (shortest dimension) of the tumour. Moribund animals were killed according to the protocols of the University of Pennsylvania. Tumour growth rates in the xenograft experiment were evaluated by fitting a linear mixed effects model on the log 10 -transformed tumour volume with days, experiment indicator (MSI short hairpin RNA (shRNA) versus control shRNA) and interaction between days and experiment included as independent variables. TOPFlash assays TOP/FOPFlash assays were carried out using the Dual-Luciferase Reporter Assay System (Promega), 293 cells were seeded in 24-well plate 12 h before co-transfection with 1,200 ng scrambled hairpin, Sh-MSI2, Sh-BCAT or pcDNA-MSI2 and 400 ng M50 Super 8 × TOPflash or M50 Super 8 × FOPflash reporter plasmids per well (Addgene plasmids 12456 and 12457). FugeneHD was used to mediate co-transfection, and the media contained 3 nM CHIR99021 GSK3β inhibitor to insure Wnt pathway activation. The Renilla luciferase reporter vector pRL-SV40 (200 ng) was simultaneously transfected as the control for Firefly luciferase in TOP/FOP vectors. Cells were harvested 48 h after transfection. Experiments were performed at least twice with n =4 wells as technical replicates in each experiment. Western blots Cells were lysed in RIPA buffer with protease inhibitors (Roche). After quantification using a BCA protein assay kit (Pierce), 40 μg of total protein was separated with 10% SDS–PAGE under denaturing conditions and were transferred to polyvinylidene difluoride membranes (GE Healthcare). The membranes were blocked in 5% BSA (Sigma) and then incubated with a Msi2 primary antibody (1:1,000; Novus Biologicals), Msi1 (1:1,000; MBL), Notch intracellular domain (1:1,000; Abcam), Hes1 (1:1,000; Abcam), β-actin (1:10,000; Abcam), Pten (1:1,000; Cell Signaling) or APC (1:200; Santa Cruz sc-896) followed by incubation with a secondary antibody conjugated with horseradish peroxidase (HRP; 1:2,000; Cell Signaling) together with an HRP-conjugated primary antibody for β-actin (1:10,000; Sigma). Immunoreactive proteins were visualized using LumiGLO chemiluminescent substrate (Pierce). Raw scans of western blots in Figs 4c , 5c , 6f and 7a can be found in the Supplementary Information accompanying the manuscript. Accession codes: CLIP-Seq data are publicly available in the NCBI GEO repository, accession number GSE64388 . Transcriptome profiling data are publicly available in the NCBI GEO repository, accession number GSE64643 . How to cite this article: Wang, S. et al. Transformation of the intestinal epithelium by the MSI2 RNA-binding protein. Nat. Commun. 6:6517 doi: 10.1038/ncomms7517 (2015).